Probing the nature of gold–carbon bonding in gold–alkynyl complexes Homogeneous catalysis by gold involves organogold complexes as precatalysts and reaction intermediates. Fundamental knowledge of the gold–carbon bonding is critical to understanding the catalytic mechanisms. However, limited spectroscopic information is available about organogolds that are relevant to gold catalysts. Here we report an investigation of the gold–carbon bonding in gold(I)–alkynyl complexes using photoelectron spectroscopy and theoretical calculations. We find that the gold–carbon bond in the ClAu–CCH − complex represents one of the strongest gold–ligand bonds—even stronger than the known gold–carbon multiple bonds, revealing an inverse correlation between bond strength and bond order. The gold–carbon bond in LAuCCH − is found to depend on the ancillary ligands and becomes stronger for more electronegative ligands. The strong gold–carbon bond underlies the catalytic aptness of gold complexes for the facile formation of terminal alkynyl–gold intermediates and activation of the carbon–carbon triple bond. Homogeneous catalysis by gold complexes has been undergoing a remarkable development over the past decade, in particular, for alkyne activation [1] , [2] , [3] , [4] , [5] , [6] , [7] . Numerous reaction intermediates have been proposed, but in general it is a challenge to directly observe and characterize these transient species. Clearly, the nature of the bonding between the Au centre and its substrates is critical to the understanding of the mechanisms of homogeneous gold catalysis. Well-defined gold complexes can serve as model systems to probe the Au-substrate bonding. However, although it is generally known that the strong relativistic effects [8] give rise to the many unique chemical properties for gold [9] , [10] , [11] , there is a scarcity of experimental studies of the Au–C bonding in organogold complexes that are most relevant to understanding the viability of catalytic intermediates and mechanisms [12] , [13] . As a powerful experimental technique to probe the electronic structure and chemical bonding of molecules, photoelectron spectroscopy has been used to study a series of Au–CN complexes recently [14] , [15] but has not been applied to any organogold complexes. Here we present the first photoelectron spectroscopy investigation of a series of Au(I)–alkynyl complexes, LAuCCH − (L=Cl, I, CCH), accompanied by ab initio calculations, to probe the nature of the Au–C bonding. Vibrationally resolved photoelectron spectra suggest that the Au–C bonding in LAuCCH − is extremely strong. Theoretical calculations show that the Au–C bond in ClAu–CCH − is one of the strongest known gold bond with a dissociation energy of 5.01 eV. Further theoretical studies find that the Au–C single bond in ClAuCCH − is even stronger than the known Au=C double bond in ClAu=CH 2 and the Au≡C triple bond in ClAu≡C, uncovering an unprecedented inverse correlation between bond strength and bond orders for gold. Such strong LAu – C≡CH − bonding implies that the formation of terminal alkynyl–gold is thermodynamically favourable, which is known to have important roles in alkyne activation. Photoelectron spectroscopy We produced the LAuCCH − complexes (L=Cl, I, CCH) by electrospray ionization of an acetonitrile solution dissolved with HC≡C–MgCl and gold iodide. The photoelectron spectra were obtained for these Au(I) complexes at various temperatures and several detachment laser wavelengths. 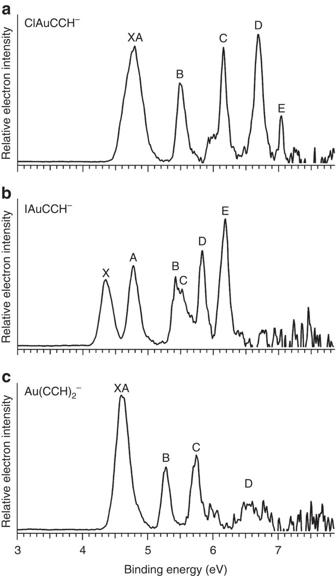Figure 1: Photoelectron spectroscopy. Measurements performed at 157 nm and room temperature for (a) ClAuCCH–, (b) IAuCCH–and (c) Au(CCH)2. Figure 1 presents the room temperature spectra of LAuCCH − (L=Cl, I, CCH) measured at 157 nm. Higher-resolution spectra for the low-binding energy features were obtained at lower photon energies (245 and 266 nm) for vibrationally cold anions at 20 K, as shown in Fig. 2 . Figure 1: Photoelectron spectroscopy. Measurements performed at 157 nm and room temperature for ( a ) ClAuCCH – , ( b ) IAuCCH – and ( c ) Au(CCH) 2 . 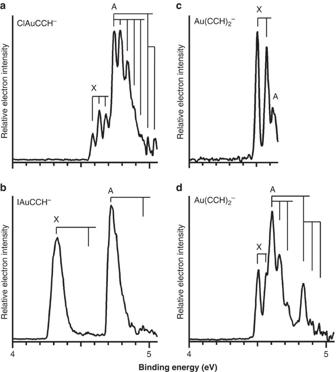Figure 2: Photoelectron spectroscopy at 20 K. (a) ClAuCCH–at 245 nm. (b) IAuCCH–at 245 nm. (c) Au(CCH)2–at 266 nm. (d) Au(CCH)2–at 245 nm. The vertical lines indicate the resolved vibrational structures. Full size image Figure 2: Photoelectron spectroscopy at 20 K. ( a ) ClAuCCH – at 245 nm. ( b ) IAuCCH – at 245 nm. ( c ) Au(CCH) 2 – at 266 nm. ( d ) Au(CCH) 2 – at 245 nm. The vertical lines indicate the resolved vibrational structures. Full size image The 157-nm spectrum of ClAuCCH − displays six major detachment bands labelled with letters (X, A–E; Fig. 1a ). The X and A bands are vibrationally resolved in the 20 K spectrum at 245 nm ( Fig. 2a ). The observed vibrational frequency of the X band (380 cm −1 ) corresponds to the ClAu stretching mode in the neutral ground state of ClAuCCH. Two vibrational progressions are resolved in the A band: a low-frequency mode of 360 cm −1 mainly corresponding to ClAu stretching and a high-frequency mode of 1960, cm −1 , which should be due to the C≡C stretching. The 157-nm spectrum of IAuCCH − also exhibits six major detachment bands ( Fig. 1b ). For the 245-nm spectrum of IAuCCH − at 20 K ( Fig. 2b ), only a very short progression of the C≡C stretching mode with a frequency of 1,860 cm −1 is discernible for the X and A bands. The relatively broad peak widths of the X and A bands suggest that there are unresolved low-frequency vibrational excitations, most probably because of the low-frequency I–Au stretching, similar to the ClAu stretching observed in the ClAuCCH − spectrum. The 157-nm spectrum of Au(CCH) 2 − reveals five major detachment bands ( Fig. 1c ), where the X and A bands overlap and the D band is weak and broad. For Au(CCH) 2 − at 20 K, spectra are taken at both 266 nm ( Fig. 2c ) and 245 nm ( Fig. 2d ). A vibrational progression with a frequency of 480 cm −1 is observed for the X band, corresponding to the Au–C stretching mode in the neutral Au(CCH) 2 ground state. Two vibrational progressions are observed for the A band ( Fig. 2d ) with frequencies of 450 and 1,850 cm −1 , respectively. The lower frequency mode should be due to the Au–C stretching and the higher-frequency mode due to the C≡C stretching in the first excited state of neutral Au(CCH) 2 . The spectral features and vibrational structures for Au(CCH) 2 − are similar to those for ClAuCCH − . The adiabatic detachment energies (ADEs), vertical detachment energies (VDEs) and the resolved vibrational frequencies of the X and A bands for all three complexes are summarized in Table 1 , where they are compared with the theoretical calculations. The VDEs and assignments for all the observed features are given in Supplementary Table S1 . We note that the Au–C vibrational frequency observed in the spectra of Au(CCH) 2 − is larger than the Au–C frequency observed in the photoelectron spectra of Au(CN) 2 − reported previously (400 cm −1 ) [14] . This observation is surprising, suggesting that that Au–CCH bond may be even stronger than the Au–CN bond in their corresponding neutral ground states. Table 1 Detachment energies and vibrational frequencies. Full size table Quantum chemical calculations and spectral interpretation High-level theoretical calculations were performed for the three Au(I) complexes and their corresponding neutrals using both density functional theory (DFT) and ab initio wavefunction theory. The optimized geometries for the three complexes are all linear in both charge states, as shown in Supplementary Table S2 , where all bond lengths are given at two levels of theory. 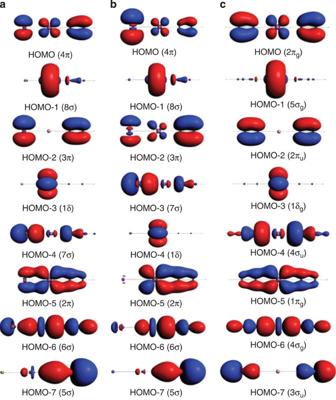Figure 3: MO analyses. MO isosurfaces (isocontour=0.05 a.u.) from ADF/B3LYP/TZ2P calculations (see Methods) for (a) ClAuCCH–, (b) IAuCCH–and (c) Au(CCH)2. HOMO, highest occupied MO. Figure 3 shows the isocontour surfaces of the Kohn–Sham molecular orbitals (MOs) of LAuCCH − . When spin-orbit (SO) coupling effects are included, the π- and δ-orbitals split into two levels, as illustrated qualitatively in Supplementary Fig. S1 . The valence MOs and electronic structures of all three complexes are similar ( Fig. 3 ). The highest occupied MO (HOMO) is of π-symmetry, consisting of antibonding combinations between the Au d π orbitals and CCH π-bonding orbital (and halogen p π orbitals for ClAuCCH − and IAuCCH − ). The SO splitting gives rise to the 2 Π 3/2 ground state and the 2 Π 1/2 first excited state for neutral LAuCCH, corresponding to the X and A bands in the photoelectron spectra ( Fig. 2 ), respectively. The calculated ADEs and VDEs are compared with the experimental observations in Table 1 for the X and A bands and Supplementary Table S1 for all observed transitions. The calculations at the CCSD(T) level without SO corrections appear to overestimate the ADEs and VDEs by ~0.1−0.3 eV relative to the experimental data. Because of the contribution of the halogen p π orbital to the HOMO, the SO splitting is the largest in IAuCCH among the three complexes. The simulated spectra using the calculated VDEs are given in Supplementary Fig. S2 , which are in qualitative agreement with the experimental spectra shown in Fig. 1 . Vibrational frequencies for the neutral ground state of LAuCCH are calculated ( Supplementary Table S3 ) and confirm the assignments of the observed vibrational structures. In particular, the calculated Au–C vibrational frequency (476 cm −1 ) for Au(CCH) 2 agrees well with the observed frequency of 480 cm −1 . The calculated Au–C stretching is 492 cm −1 for ClAuCCH and 473 cm −1 for IAuCCH, consistent with the strong Au–C bonding. Figure 3: MO analyses. MO isosurfaces (isocontour=0.05 a.u.) from ADF/B3LYP/TZ2P calculations (see Methods) for ( a ) ClAuCCH – , ( b ) IAuCCH – and ( c ) Au(CCH) 2 . HOMO, highest occupied MO. Full size image Unusually strong and L-dependent Au–C bond in LAuCCH − As shown in Fig. 3 , the HOMO-5 for the three Au(I) complexes is a strong π-bonding orbital, whereas the HOMO is an antibonding π-orbital. Thus, there is no net π-bonding between Au and the CCH ligand. The Au–CCH bonding comes mainly from HOMO-6, which is a σ-MO from the overlap of the Au 5 d z 2 and the sp hybrid orbital on CCH. The Au–CCH interaction can be characterized by a single σ-bond, as supported by the bond order analyses ( Table 2 ) [16] . This bonding picture is consistent with the fact that the alkynyl ligand is known to be a good σ- and π-donor but a poor π-acceptor because of the high energy of its antibonding π*-orbitals [17] , [18] , [19] . The covalent interaction between Au and the alkynyl ligand is more clearly illustrated in the electron localization functions presented in Fig. 4 . Table 2 Bond parameters. 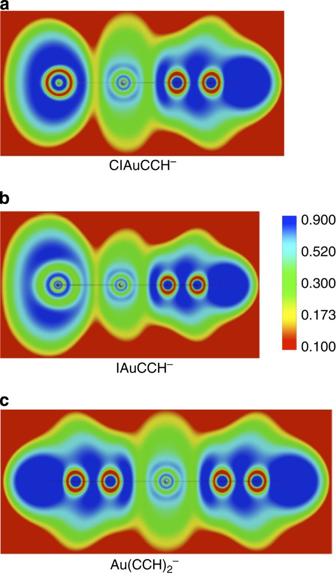Figure 4: Chemical bonding analyses. Electron localization functions (ELFs) calculated for (a) ClAuCCH–, (b) IAuCCH–and (c) Au(CCH)2. The ELF represents the probability to find electron pairs between two atoms and reveals strong covalency in the Au–C bond. Full size table Figure 4: Chemical bonding analyses. Electron localization functions (ELFs) calculated for ( a ) ClAuCCH – , ( b ) IAuCCH – and ( c ) Au(CCH) 2 . The ELF represents the probability to find electron pairs between two atoms and reveals strong covalency in the Au–C bond. Full size image However, the strong Au–C stretching vibrational frequency of 480 cm −1 observed in the photoelectron spectrum of Au(CCH) 2 − in Fig. 2 suggests that the Au–C bond is unusually strong in the neutral Au(CCH) 2 ground state. This frequency is >400 cm −1 frequency observed for the Au–C stretching in the photoelectron spectrum [14] of Au(CN) 2 − , a well-known and highly stable Au(I) complex used to extract gold for centuries [20] . This observation led us to suspect that the Au–CCH bonding might also be stronger than the Au–CN bonding in their respective anionic complexes. We calculated the dissociation energy of AuX 2 − →Au + +2X − at the ADF/PBE level (see Methods) and found that indeed this quantity for X=CCH (15.07 eV) is higher than that for X=CN (14.62 eV). We further calculated the bond dissociation energy ( D e ) for LAu–CCH − →LAu+CCH − and found that D e strongly depends on the ligand L ( Supplementary Table S4 ); the D e for L=Cl is significantly higher than that for L=HCC and I. This is known as the trans -effects [18] , [19] . The more electronegative L ligands polarize the Au(I) centre and strongly enhance the Au–C bond in LAu–CCH – . We subsequently calculated the D e for a series of Au(I) complexes, as given in Supplementary Table S4 . Except for FAu–CCH – and ClAuCH 3 – , the D e of ClAu–CCH – is the highest. The D e shown in Supplementary Table S4 represents heterolytic bond cleavage processes, producing two closed shell and stable fragments. Heterolytic bond cleavages are usually used when considering the bonding in donor–acceptor-type complexes [21] . We further computed the heterolytic D e of ClAuCCH – , ClAuCN – and ClAuCH 3 – at the CCSD(T)/AVTZ level and obtained 5.01, 4.52 and 5.64 eV, respectively ( Supplementary Table S5 ), which are similar to those at the DFT level ( Supplementary Table S4 ). We also computed the homolytic dissociation energies for ClAu–CCH – , ClAuCN – and ClAuCH 3 – to produce two open shell species: ClAu – and a radical ·CCH, ·CN and ·CH 3 , respectively, as 5.83, 6.23 and 3.52 eV at the CCSD(T) level ( Supplementary Table S5 ). To eliminate possible charge effects, we further considered the D e of the three neutral complexes, ClAuCCH (→ ClAu+·CCH), ClAuCN (→ ClAu+·CN) and ClAuCH 3 (→ ClAu+·CH 3 ), which can be viewed to consist of a one-electron Au–C bond. The D e of ClAu–CCH is the highest among the three species with a value of 3.19 eV, which would yield an estimated 6.32 eV for a two-electron Au–C bond, comparable to the 5.01 eV donor–acceptor bond energy. Interestingly, the D e of ClAuCH 3 →ClAu+·CH 3 is very low, only 1.33 eV, suggesting a strong charge effect in the donor–acceptor interaction in the ClAuCH 3 – anionic complex. These analyses suggest that the ClAuCCH – complex represents one of the strongest Au–C bonds. The donor–acceptor D e of 5.01 eV for ClAu–CCH – at the CCSD(T) level is an extremely high bond energy, even higher than that of ClAuCN – by ~0.5 eV ( Table 2 and Supplementary Table S5 ). Inverse correlation between bond order and bond strength To understand the nature of the strong Au–C bond in ClAu–CCH – , we compare it with the multiple Au–C bonds in Table 2 . It is known that Au forms a double bond with carbene [22] , [23] in [Au=CH 2 ] + and a triple bond [24] , [25] with C in [Au≡C] + . The neutral forms of the species containing the multiple Au–C bonds have been studied by complexing with halogen counter ions [26] , [27] . We have calculated the bond lengths and D e for the Au–C double bond in ClAu=CH 2 and triple bond in ClAu≡C, and have compared them with those of ClAu–CCH – in Table 2 , which also lists literature values for [Au=CH 2 ] + and [Au≡C] + . The isosurfaces of the MOs of ClAu=CH 2 and ClC≡Au are given in Supplementary Fig. S3 , from which one can get a glimpse of the multiple bond nature of these two molecules. The data in Table 2 reveal remarkably that the Au–C single bond in ClAu–CCH – is even stronger than the Au=C and Au≡C multiple bonds, although the bond lengths of the multiple bonds are shorter. The Au=C and Au≡C multiple bonds were suggested in previous theoretical studies on the bases of the short Au – C bond lengths and MO analyses (also see Supplementary Fig. S3 ) [22] , [23] , [24] , [25] , [26] , [27] . The current bond-order analyses generally support the formal bond-order designations ( Table 2 ), although the numerical values are usually smaller [28] . It is interesting to note that the Cl – complexation in ClAu=CH 2 and ClAu≡C slightly weakens the Au–C multiple bonds, whereas it strengthens the Au–C single bond in ClAu–CCH – . The Au–C bond length decreases with increasing bond order from the single bond in ClAu–CCH – to the double bond in ClAu=CH 2 , and the triple bond in ClAu≡C. However, the D e of the single Au–C bond in ClAu–CCH – is about 1.5 eV higher than that of the Au=C double bond in ClAu=CH 2 , which in turn is stronger by about 0.2 eV than the Au≡C triple bond in ClAu≡C ( Table 2 ). This remarkable inverse correlation between bond strength and bond order/bond length is unprecedented for gold. The breakdown of bond strength and bond length correlation has been seen in F-substituted ethane or other heavier group-14 species, such as in C 2 H 6− n F n or Sn 2 H 6− n F n , mainly because of the Pauli repulsion of the inner-shell electrons between the heavier elements [29] , [30] , [31] , [32] . Inverse correlation of bond strength and bond order is very rare. A weak inverse correlation between bond order and bond strength is known in CH 2 =XH 2 (X=Si, Ge, Sn and Pb) and some metal–metal multiple bonded species [29] , [33] . The inverse correlation between bond order and bond strength in the Au–C species can be attributed to the strong relativistic effects of Au, which result in extremely short double and triple bond lengths, leading to strong Pauli repulsion between the inner-shell electrons of Au and C. The Au–C bond in the LAu–CCH – complexes (L=Cl, I, CCH) is shown here to be one of the strongest Au–ligand bond known. The ancillary ligand is found to strongly influence the strength of the Au–C bond, consistent with the fact that the catalytic efficiency of LAu(I) complexes is highly dependent on the nature of L. The strong Au–C bond in Au(I) alkynyl complexes weakens and activates the C≡C triple bond and prepares it for the subsequent C–C coupling reactions. The remarkable inverse correlation between bond order and bond strength in the Au–C complexes underlies the strength of the Au–alkynyl bond and furthers our understanding of the expanding gold chemistry. Experiments The experiment was done using a magnetic-bottle photoelectron spectroscopy apparatus equipped with an electrospray ionization source [34] and a cryogenically cooled ion trap [35] . The LAuCCH − (L=Cl, I, CCH) complexes were prepared by electrospray of an acetonitrile solution dissolved with the Grignard-type HCC–MgCl compound and gold iodide. The electrospray source was purged with a flow of N 2 gas and the produced anions were accumulated in a Paul trap operated both at room temperature and low temperatures [36] . The desired anion was mass selected by a time-of-flight mass spectrometer. Photoelectron spectra were obtained using three detachment lasers, 157 nm from an F 2 excimer laser, 245 nm from a dye laser and 266 nm from a Nd:YAG laser. The experiment was calibrated by the known spectra of Au − and I − . The electron kinetic energy resolution of the current magnetic-bottle photoelectron analyser was about Δ E / E =3%, that is, 30 meV for 1 eV electrons. Theory and computation The calculations were performed using DFT and ab initio wavefunction theory. The DFT calculations were done using the generalized gradient approximation with PBE exchange-correlation functional [37] and hybrid B3LYP functional [38] , [39] as implemented in the Amsterdam Density Functional program (ADF 2010.01) [40] . The Slater basis sets with the quality of triple-ζ plus two polarization functions (TZ2P) with the frozen core approximation applied to inner shells were used. The scalar relativistic (SR) and SO coupling effects were taken into account by the zero-order-regular approximation (ZORA) [41] . Geometries were fully optimized at the SR-ZORA level and single-point energy calculations were performed with the inclusion of the SO effects. Vibrational frequency calculations were carried out at the SR-ZORA level with PBE functional. To confirm the ADE and the first VDE (VDE 1 ), high-level CCSD(T) single-point energy calculations were performed using the MOLPRO 2008 program [42] at the B3LYP-optimized geometries from Gaussian 09 (ref. 43 ). In the MOLPRO and Gaussian 09 calculations, the aug-cc-pVTZ basis set was used for all atoms [44] , [45] except the cc-pVTZ-PP basis set for Au [46] and I [47] , and the Stuttgart SR effective core potential was used for heavier elements I [47] and Au [48] . The optimized geometries for anionic and neutral LAuCCH (L=Cl, I, CCH) are all linear ( Supplementary Table S2 ), and are confirmed as minima through frequency analyses at the DFT level with PBE and B3LYP functionals. The calculated VDEs ( Supplementary Table S1 ) were obtained using generalized Koopmans’s theorem by aligning the VDE 1 with the experimental value [49] . The ADE and VDE 1 were also calculated using the single-point CCSD(T) [50] calculations with the B3LYP-optimized geometries ( Table 1 ). How to cite this article: Liu, H.-T. et al. Probing the nature of gold–carbon bonding in gold–alkynyl complexes. Nat. Commun. 4:2223 doi: 10.1038/ncomms3223 (2013)